Synthesis of hexagonal close-packed gold nanostructures Solid gold is usually most stable as a face-centred cubic ( fcc ) structure. To date, no one has synthesized a colloidal form of Au that is exclusively hexagonal close-packed ( hcp ) and stable under ambient conditions. Here we report the first in situ synthesis of dispersible hcp Au square sheets on graphene oxide sheets, which exhibit an edge length of 200–500 nm and a thickness of ~ 2.4 nm (~ 16 Au atomic layers). Interestingly, the Au square sheet transforms from hcp to a fcc structure on exposure to an electron beam during transmission electron microscopy analysis. In addition, as the square sheet grows thicker (from ~ 2.4 to 6 nm), fcc segments begin to appear. A detailed experimental analysis of these structures shows that for structures with ultrasmall dimensions (for example, <~ 6 nm thickness for the square sheets), the previously unobserved pure hcp structure becomes stable and isolable. Anisotropic noble metal nanoparticles (gold (Au) and silver (Ag)) are a class of materials with chemical and physical properties that directly correlate with their structures. They have been used for many applications in biosensing, intracellular gene regulation, photonics and catalysis [1] , [2] , [3] , [4] , [5] . Colloids of well-dispersed spherical Au nanoparticles were successfully synthesized decades ago by refluxing HAuCl 4 with sodium citrate [6] . These procedures have been refined, and now can reliably be used to prepare monodisperse samples of particles in the 2- to 200-nm diameter range. In addition to particle size control, particle shape control is also important. Over the past 10 years, significant strides have been made in synthesizing anisotropic Au nanostructures (AuNSs) [7] , [8] , [9] . To realize anisotropic growth, template-mediated syntheses are some of the most effective approaches. Examples include the surfactant-directed soft-templating method [7] and the biomolecule-facilitated hard-templating approach [10] . More recently, ultrathin single-crystalline Au nanowires (AuNWs) were synthesized by slow reduction of HAuCl 4 in the presence of 1-amino-9-octadecene, which serves as a soft template for the growth of the wires [5] , [11] , [12] . Graphene, a single atomic layer of graphite, has attracted tremendous attention because of its exceptional physical properties and promise in various applications [13] , [14] . One of its derivatives, graphene oxide (GO), is an extensively oxidized two-dimensional (2D) carbon sheet, which is suitable for chemical modification and subsequent device incorporation [15] . These structures also have interesting properties. To date, researchers have used them to synthesize nanoparticles, but the resulting structures have been mostly spherical [16] or lack good crystallinity [17] . Herein, we report the in situ synthesis of pure hexagonal close-packed ( hcp ) Au square sheets (AuSSs) on GO. The AuSSs, with an edge length of 200–500 nm and a thickness of ~ 2.4 nm (~ 16 Au atomic layers), consist of a unique atomic arrangement of Au. A detailed experimental analysis of this structure shows that for a structure with ultrasmall dimensions (for example, less than ~ 6-nm thickness for the AuSSs), the pure hcp phase becomes stable and isolable at ambient conditions. In addition, we show that the crystal lattice of the AuSSs transforms from the hcp phase to a face-centred cubic ( fcc ) structure on exposure to a transmission electron microscope (TEM) beam. Synthesis and characterization of AuSSs The AuSSs were synthesized by heating a solution containing GO sheets, 4-mM HAuCl 4 and 140-mM 1-amino-9-octadecene, CH 3 (CH 2 ) 7 CH=CH(CH 2 ) 8 NH 2 , in a solution of hexane and ethanol (v/v=23:2) at 55 °C for 16 h ( Supplementary Fig. S1 ). Interestingly, the obtained pseudo-square-shaped nanostructures exhibit an edge length between 200 and 500 nm, as determined by TEM analysis ( Fig. 1a ). The Au composition of the as-prepared nanostructures was confirmed by energy dispersive X-ray analysis ( Supplementary Fig. S2 ). The thickness of a typical AuSS, which is estimated by measuring the width of folded edges of an AuSS ( Supplementary Fig. S3 ), is 2.4±0.7 nm. Note that a similar method has been used to characterize monolayer and bilayer sheets of graphene [13] . Atomic force microscopy measurements for a typical AuSS on GO ( Supplementary Fig. S4 ) indicate a thickness of 4 nm, which is ~ 1.6 nm greater than the thickness of the AuSS core, as determined by TEM. This apparent increase in thickness is because the alkylamine molecules, adsorbed on the AuSS surface [18] , are invisible by TEM but are clearly present based on X-ray photoelectron spectroscopy ( Supplementary Fig. S5 ). Surprisingly, these AuSSs are hcp (2H type) nanostructures, as evidenced by selected area electron diffraction (SAED) data ( Fig. 1c,d ). For example, a typical AuSS oriented on GO, with its square basal plane normal to the electron beam (e-beam), exhibits two rings assigned to the GO {100} and {110} planes with lattice spacings of 2.2 and 1.3 Å, respectively ( Fig. 1c ; note that directly dropping the sample solution onto a copper grid often results in multilayer GO deposition). The remaining diffraction spots for the AuSS fit the hcp Au lattice structure (2H type, with a symmetry of P63/mmc), viewed along the [110] h direction. The SAED pattern taken at [320] h zone axis ( Fig. 1d ) was also obtained by tilting an AuSS along the (1[macr1]1) h reflection by ~ 19° with respect to the [110] h zone axis, in agreement with the theoretical angle between [320] h and [110] h , that is, 19°. For further comparison and confirmation, SAED patterns along the [110] h and [320] h zone axes were simulated ( Supplementary Fig. S6 ), which are consistent with the patterns obtained experimentally ( Fig. 1c,d ). X-ray diffraction (XRD) data for AuSSs on GO, deposited on a glass slide, are also consistent with the hcp assignment ( Supplementary Fig. S7 ). The peaks at ~ 37 and ~ 40° are associated with the Au (002) h and (101) h planes, respectively, for a 2H- hcp phase (the simulated unit cell parameters are a =2.96 Å and c =4.84 Å). The remaining peaks are from fcc Au, because of the presence of spherical Au nanoparticles (byproducts of the reaction forming the AuSSs, see the several dark Au dots with size of 10–25 nm in Fig. 1a ). Note that the peaks for hcp phase appear very weak as compared with the fcc phase. This observation, in part, is because of their anisotropic properties. The AuSSs on GO sheets deposited on a substrate for XRD were so highly oriented that not all of the crystal planes showed strong reflections; however, the pseudo-spherical fcc Au nanoparticles were randomly distributed on the substrate, giving rise to the strong reflections from different crystal planes ( Supplementary Fig. S7a ). In addition, the reflections from the (110) h square basal planes of AuSSs are barely observable because of the ultrathin nature of the AuSSs. The 2.4-nm dimension, normal to the (110) h plane, results in a weak and broad reflection peak based on Sherrer's theory [19] , whereas the fcc Au nanoparticles, which are 10–25 nm in diameter, produce strong reflections. For comparison, a concentrated solution (similar to a paste) of AuSSs was deposited on a glass slide, so that the AuSSs did not show the preferred orientation. As a result, stronger signals for hcp phase, for example, those for the (002) h and (101) h planes, were observed with considerable broadening and overlapping ( Supplementary Fig. S7b ). The high-resolution TEM (HRTEM) image of a small section of a typical AuSS matches the lattice pattern of a 2H- hcp Au along the [110] h zone axis ( Fig. 1b ). A series of simulated HRTEM images of hcp Au sheets, which vary in thickness, are shown in Supplementary Figure S8 . 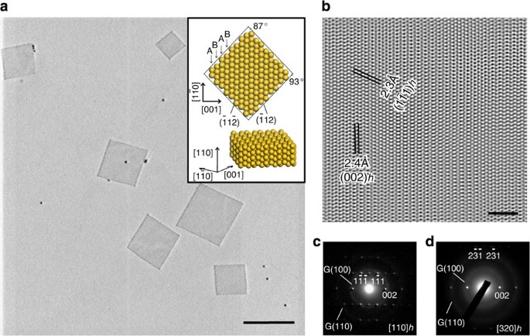Figure 1: TEM analysis of Au square sheets. (a) TEM image of ~ 2.4-nm thick AuSSs on a GO surface (scale bar, 500 nm). The black dots are nanoparticle byproducts, that is, spherical Au nanoparticles (approximately 10–25 nm).Inset: crystallographic models for a typical AuSS with its basal plane along the [110]hzone axis, showing ABAB stacking along the [001]hdirection. (b) HRTEM image of a small region of a typical AuSS oriented normal to [110]h, as indicated from the SAED inc(scale bar, 2 nm). (c) SAED pattern of an AuSS on GO sheets, showing diffraction rings for GO and spots for [110]hzone axis of the AuSS. (d) SAED of [320]hzone axis was collected by tilting an AuSS from the [110]hzone axis along the (1[macr1]0)hreflection by~ 19°. The calculated lattice spacings for (002) h and (1[macr1]1) h based on the XRD results are 2.42 and 2.27 Å, respectively, which are in agreement with the measured values in the HRTEM image of the AuSS, Figure 1b . The calculated lattice spacing for the (110) h basal planes is 1.48 Å; thus, an AuSS with a thickness of 2.4 nm contains ~ 16 Au atomic layers. The AuSSs are not perfect squares. The two opposite angles along the [002] h diagonal (93°) are slightly larger than those along the [1[macr1]0] h diagonal (87°), which matches well with the interplane angles of (1[macr1]2) h /([macr1]12) h (93.3°) and ([macr1]1[macr2]) h /([macr1]12) h (86.7°), respectively. Therefore, crystal models, with 2D and 3D views, for the AuSSs are proposed in the inset of Figure 1a , indicating that the square basal plane in each nanostructure is normal to the [110] h direction, with ABAB stacking along the [001] h direction, and four sides enclosed by {[macr1]12} h planes. Figure 1: TEM analysis of Au square sheets. ( a ) TEM image of ~ 2.4-nm thick AuSSs on a GO surface (scale bar, 500 nm). The black dots are nanoparticle byproducts, that is, spherical Au nanoparticles (approximately 10–25 nm). Inset : crystallographic models for a typical AuSS with its basal plane along the [110] h zone axis, showing ABAB stacking along the [001] h direction. ( b ) HRTEM image of a small region of a typical AuSS oriented normal to [110] h , as indicated from the SAED in c (scale bar, 2 nm). ( c ) SAED pattern of an AuSS on GO sheets, showing diffraction rings for GO and spots for [110] h zone axis of the AuSS. ( d ) SAED of [320] h zone axis was collected by tilting an AuSS from the [110] h zone axis along the (1[macr1]0) h reflection by~ 19°. Full size image When the aforementioned growth solution for the AuSSs on GO was heated at 55 °C for 28 h, the AuSSs became thicker (6.0±0.7 nm, Supplementary Fig. S9b ), but exhibit a similar square-like shape with truncated corners ( Supplementary Fig. S9 ). Alternating dark and bright strips are observed along one of the diagonals ( Supplementary Fig. S9a ), indicating the presence of stacking faults or twin defects. Indeed, HRTEM images and XRD pattern confirm the mixed stacking of hcp and fcc planes ( Supplementary Figs. S7c and S9c ), suggesting that as the AuSS grows thicker (from about 2.4 to 6.0 nm) the pure hcp phase becomes less stable. Although AuSSs can be synthesized without GO sheets by heating a mixture of HAuCl 4 , 1-amino-9-octadecene, hexane and ethanol, the resulting AuSSs have a large size distribution (30–500 nm), with the coexistence of AuNWs and Au nanoparticles ( Supplementary Fig. S10 ). Indeed, the yield, uniformity and quality of the AuSSs are greatly enhanced when they are synthesized in situ on the GO sheets. The synthesis of AuSSs requires a mixed solvent of ethanol and hexane, whereas the synthesis of AuNWs uses pure hexane as the solvent [12] . We believe that the solvent polarity may have a critical effect on the morphology of 1-amino-9-octadecene–AuCl complex, for example, the square-shaped complex shown in the synthesis of AuSSs ( Supplementary Fig. S11 ). The GO sheet contains the abundant oxygenated functional groups, which increases the polarity at its proximity and thus suppresses formation of AuNWs. E-beam-induced hcp – fcc phase transformation of AuSSs The hcp to fcc phase transformation of an AuSS was observed during TEM analysis. We found that a HRTEM image of pristine hcp phase could only be captured within a very short period of time (<5 s). More detailed studies showed that when an AuSS was irradiated with an e-beam for ~ 20 s, the AuSS gradually became porous ( Fig. 2a,b ), which was similarly observed by others in the melting and splitting of ultrathin AuNWs during TEM characterization [12] . This porous AuSS yields a SAED pattern consistent with the formation of the twinned fcc phase when viewed along the [101] f zone axis ( Fig. 2c ). Reflection spots resulting from twinning are observed and denoted with a subscript 'T' ( Fig. 2c ). A lattice spacing of 2.4 Å is measured along one of the diagonals of the porous AuSS, corresponding to the fcc (111) planes. Such structures with a high density of twinning and stacking faults are commonly observed in semiconductor nanowires [20] and recently reported Ag rod–needle heterogeneous structures [21] . 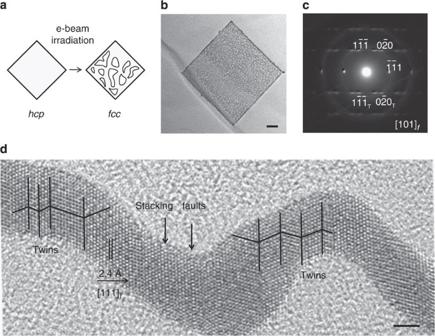Figure 2: Images illustrating the e-beam-induced phase transformation of Au square sheet. (a) Scheme of the e-beam-induced phase transformation of an AuSS. (b) TEM image of a porous AuSS after e-beam irradiation for ~ 20 s (scale bar, 50 nm). (c) SAED pattern of a porous AuSS after e-beam irradiation, showing the twinned structure viewed along the [101]fdirection. (d) HRTEM image of a section of a porous AuSS, with marked twins and stacking faults (scale bar, 2 nm). Figure 2: Images illustrating the e-beam-induced phase transformation of Au square sheet. ( a ) Scheme of the e-beam-induced phase transformation of an AuSS. ( b ) TEM image of a porous AuSS after e-beam irradiation for ~ 20 s (scale bar, 50 nm). ( c ) SAED pattern of a porous AuSS after e-beam irradiation, showing the twinned structure viewed along the [101] f direction. ( d ) HRTEM image of a section of a porous AuSS, with marked twins and stacking faults (scale bar, 2 nm). Full size image To further investigate the phase transformation process, a series of in situ time-dependent HRTEM images were taken ( Supplementary Fig. S12 ). During the initial 20-s irradiation period, small domains of fcc packing (marked in red rectangles) begin to appear within what originally was a pure hcp structure ( Supplementary Figs. S12a,b ). After Irradiation for another 20 s, the long-range order of the hcp lattice was interrupted, and the lattice structure becomes distorted over the entire area ( Supplementary Fig. S12c ), a consequence of a significant rearrangement of the Au atoms. After irradiation for 60 s, the fcc structure became dominant with some defect areas (dotted red rectangle, Supplementary Fig. S12d ). When the irradiation time is 150 s, the defect regions continue to transform to the fcc structure ( Supplementary Fig. S12e ), and eventually an fcc lattice with stacking faults and twin defects was formed ( Supplementary Fig. S12f ). The hcp to fcc phase transformation of the AuSS is believed to be due to the high-energy e-beam. As reported previously [22] , the temperature of an e-beam irradiated structure can be as high as 500 °C, resulting in thermal annealing of a nanostructure [23] . In addition, the amine molecules capped on the AuSS surface are likely removed, when the AuSS is exposed to such high energy, leaving the ultrathin Au structure unstable. As the quasi-liquid metal re-equilibrates, the Au atoms tend to transform from the hcp structure to the more stable fcc structure. This process is analogous to the e-beam irradiation-induced phase transitions observed in 3-nm ruthenium nanocrystals [24] . Note that if the total number of Au atoms remains constant, there is only slight reduction in the volume (~ 9%) due to the different phase densities; hence, the porous structure must be thicker than the flat AuSS. After the structure becomes thicker, it can be stable under e-beam irradiation without further melting. This suggests that the hcp phase is more stable in the chemically capped thinner structures. However, as the phase transformation in AuSS was not complete, the planes of hexagonal packing still exist as stacking faults and twin boundaries in the main fcc phase ( Fig. 2d ). 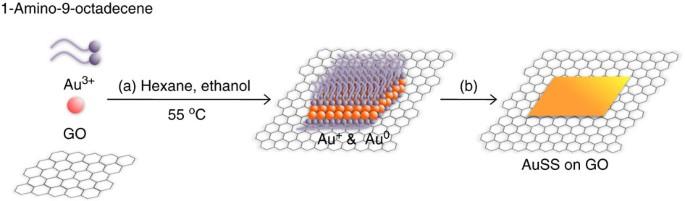Figure 3: Schematic illustration of the formation process of Au square sheet. Step (a): 1-amino-9-octadecene, Au3+and GO sheets in a mixed solvent of hexane and ethanol are heated at 55 °C. Au3+is partially reduced to Au+and complexed with 1-amino-9-octadecene.Step (b): The formed 1-amino-9-octadecene–AuCl complex, adsorbed on the GO surface, finally becomes the AuSS. Formation process of AuSSs We hypothesize that the synthesis of AuSSs on GO is facilitated by 1-amino-9-octadecene molecules ( Figure 3 ). After mixing the 1-amino-9-octadecene and Au 3+ in hexane together with GO sheets, Au 3+ is partially reduced to Au + and complexed with 1-amino-9-octadecene [11] . At the same time, the 1-amino-9-octadecene–AuCl complex adsorbs onto the GO surface because the long-chain alkylamine molecules can assist the dispersion of graphene in organic solvents [25] , which is also confirmed in our experiments. Indeed, although the GO sheets do not disperse in the pure hexane, they disperse very well in the mixed solution of 1-amino-9-octadecene (>0.1 mM) in hexane. During the synthesis of AuSSs (Step (a) in Fig. 3 ), after 8 vol% ethanol was added to the synthesis solution, which was then heated at 55 °C for ~ 8 h, the 1-amino-9-octadecene–AuCl complex was observed to self-assemble into square-like structures on the GO surface ( Supplementary Fig. S11 ). This is because the 1-amino-9-octadecene–AuCl complex can self-organize into ordered supramolecular structures through aurophilic interactions [11] , [12] , [26] , [27] . After ~ 2 h, intriguingly, small Au seeds (~ 2 nm, Fig. 4a ) begin to appear on the GO surface, and assemble into square-like assemblies. It is postulated that these Au seeds nucleate from the square-like structures formed from the 1-amino-9-octadecene–AuCl complex upon the slow reduction of Au + . The Au seeds continue to grow and fuse with one another, with a continuous supply of Au from the 1-amino-9-octadecene–AuCl complexes, resulting in the formation of dendritic Au structures with a square-like overall morphology ( Fig. 4b ). The dendritic structure, at this stage, has a high density of crystal defects, as evidenced by HRTEM image ( Fig. 4d ). Such defects are indications of the interfaces of misoriented Au nanocrystals during interparticle attachment [28] . These dendritic structures are prone to oxidative etching and smoothing, resulting in the reduction of the structure thickness, which has been reported previously in the synthesis of ultrathin AuNWs [29] , [30] . After ageing these structures for 1–2 h, the square-sheet architecture begins to reveal itself from the centre of the dendritic structure ( Fig. 4c ). 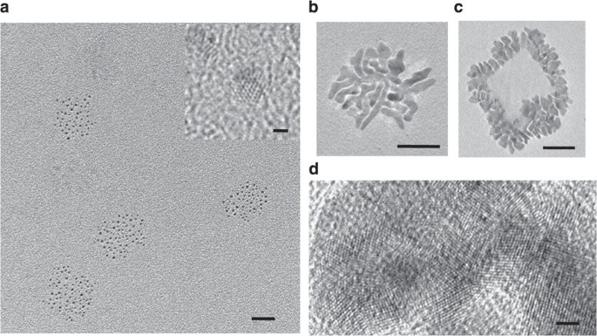Figure 4: TEM images showing the evolution of the AuSSs. (a) Small Au seeds (~ 2 nm) nucleated on the GO surface (scale bar, 20 nm),inset: an HRTEM of an Au seed (scale bar, 1 nm); (b) a dendritic Au nanostructure formed after the Au seeds fuse with one another and grow on GO (scale bar, 50 nm); (c) an Au nanostructure with the centre part showing square-sheet morphology and sides with dendritic architectures (scale bar, 50 nm); (d) HRTEM image of a section of a dendritic structure, showing the polycrystallinity (scale bar, 2 nm). The square-sheet centre is thinner than the dendritic edges based on the contrast of Figure 4c (a darkness profile is shown in Supplementary Fig. S13 ). Over time, the centre of the square structure enlarges at the expense of the side dendrites and the overall structure grows laterally, and finally a well-defined AuSS forms on the GO surface ( Fig. 1a , Step (b) in Fig. 3 ). Figure 3: Schematic illustration of the formation process of Au square sheet. Step (a) : 1-amino-9-octadecene, Au 3+ and GO sheets in a mixed solvent of hexane and ethanol are heated at 55 °C. Au 3+ is partially reduced to Au + and complexed with 1-amino-9-octadecene. Step (b) : The formed 1-amino-9-octadecene–AuCl complex, adsorbed on the GO surface, finally becomes the AuSS. Full size image Figure 4: TEM images showing the evolution of the AuSSs. ( a ) Small Au seeds (~ 2 nm) nucleated on the GO surface (scale bar, 20 nm), inset : an HRTEM of an Au seed (scale bar, 1 nm); ( b ) a dendritic Au nanostructure formed after the Au seeds fuse with one another and grow on GO (scale bar, 50 nm); ( c ) an Au nanostructure with the centre part showing square-sheet morphology and sides with dendritic architectures (scale bar, 50 nm); ( d ) HRTEM image of a section of a dendritic structure, showing the polycrystallinity (scale bar, 2 nm). Full size image A key question pertains to why the hcp phase is favoured over the fcc phase in the thin AuSSs. On the basis of the previous theoretical calculations, the fcc structure is most stable in bulk noble metals such as Ag and Au [31] , [32] , but when the dimensions of a structure are reduced to the nanometre scale, surface effects on particle and phase stability become more significant. Indeed, it has been reported that hcp (4H type) and fcc structures coexist in certain electrodeposited AgNWs [33] . In that study, the 4H-AgNW amount decreased as the diameter of AgNWs increased from 30 to 50 nm, which was confirmed by calculations showing that the 4H-phase in AgNW had a more favourable surface configuration but higher-volume internal energy than the fcc -AgNW phase [33] . Such effects have led to the realization of novel anisotropic Ag architectures with coexisting hcp and fcc phases [21] , [34] . In this contribution, the ultrathin AuSSs (thickness of ~ 2.4 nm) exhibit a similar dimensional effect, that is, the hcp phase is preferred and exclusively present in structures with at least one dimension less than 6 nm. As mentioned above, when the fcc dendritic structure undergoes oxidative etching and smoothing, the thinner square sheet appears from the centre of the structure, which grows laterally and finally becomes the hcp AuSS ( Fig. 4c ). Further, as the AuSS grows thicker from 2.4 to 6 nm, fcc segments begin to appear, resulting in the alternating hcp / fcc domains ( Supplementary Fig. S9c ). Although the hcp Au structures have been reported previously, they are not pure. For example, hcp planes are observed as crystal defects in predominantly fcc forms of Au [8] , [35] , or when a few atomic layers of Au are deposited as a film on a solid substrate [36] . Recently, hcp Au with stacking faults was observed in the catalyst used for the heterogeneous growth of germanium nanowires [37] . Under certain extreme conditions, such as ultrahigh pressure, an fcc Au can also transform to its hcp structure [38] . To the best of our knowledge, this is the first time an AuNS has been directly synthesized, which is exclusively in the hcp phase, with the unique square-sheet morphology and stable under ambient conditions. In summary, we have successfully synthesized ultrathin AuSSs that exhibit a pure hcp (2H type) phase, an unprecedented observation for a dispersible nanostructure. Our experimental observations have shown that at ultrasmall dimensions (for example, less than ~ 6-nm thickness for the AuSSs), hcp -phased Au structures are stabilized. These observations are an important fundamental advance in material science and chemistry, especially as the pure hcp AuSSs represent a new structural composition for one of the most important elements in the periodic table. Chemicals Natural graphite (SP-1) was purchased from Bay Carbon and used for synthesizing GO. Potassium permanganate (KMnO 4 ; Sigma–Aldrich), H 2 SO 4 (98%, Sigma–Aldrich), ethanol (99.9%, absolute, Merck), hexane (technique grade, Sigma–Aldrich), 1-amino-9-octadecene (CH 3 (CH 2 ) 7 CH=CH(CH 2 ) 8 NH 2 , 70%, technique grade, Sigma–Aldrich) and hydrogen tetrachloroaurate (III) (≥99.9%, Sigma–Aldrich) were used without further purification. Synthesis of GO All glassware was washed with aqua regia (HCl/HNO 3 =3:1 (v/v)), and rinsed with ultrapure water ( caution : aqua regia is a very corrosive oxidizing agent, which should be handled with great care). Graphite oxide was synthesized from natural graphite (SP-1) by the modified Hummers method [16] . The obtained graphite oxide was dispersed in water or ethanol and subsequently sonicated to yield GO. Synthesis of AuSSs on GO GO was isolated by centrifuging 0.5 ml of GO solution (0.2 mg ml −1 in ethanol) and then re-dispersed in 2 ml of growth solution containing 4-mM HAuCl 4 and 140-mM 1-amino-9-octadecene in a mixture of hexane and ethanol (v/v=23:2). The 2-ml growth solution in a 5-ml glass bottle was heated in a water bath at 55 °C for 16 h to obtain the AuSSs on GO. The final solution was centrifuged at 5,000 r.p.m. for 10 min and washed at least three times with hexane before further characterization. A small amount of solution (100 μl) was taken out at different reaction intervals to study the evolution of the synthesized AuSSs. Synthesis of AuSSs without GO AuSSs can be synthesized by using the same conditions mentioned above, without the addition of GO sheets. However, AuNWs and Au nanoparticles are also present in the obtained solution ( Supplementary Fig. S10 ). Characterization A drop of a solution containing Au nanostructures on GO sheets was placed on a holey carbon-coated copper grid, silicon, silica and glass slide, and then naturally dried in air before characterization by TEM (JEM 2010F, JEOL), Atomic Force Microscopy (Dimension 3100, Veeco), X-ray photoelectron spectroscopy (AXIS ultra spectrometer, Kratos) and X-ray diffraction (XRD, Shimadzu), respectively. How to cite this article: Huang, X. et al . Synthesis of hexagonal close-packed gold nanostructures. Nat. Commun. 2:292 doi: 10.1038/ncomms1291 (2011).